Negative cooperativity upon hydrogen bond-stabilized O2adsorption in a redox-active metal–organic framework 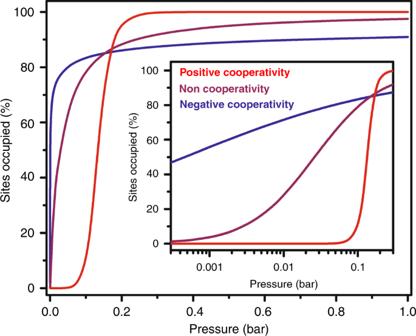Fig. 1: Illustration of adsorption isotherm variability with cooperativity. Isotherms of positively cooperative (red line), noncooperative (purple line), and negatively cooperative (blue line) systems exhibit significant differences in shape, due to the nature of the adsorbate-adsorbent interactions. In particular, negatively cooperative systems can reach half occupancy at significantly lower pressures than noncooperative and positively cooperative systems but generally require much higher pressures to reach saturation. The inset graph displays the low pressure regime (<0.2 bar) on a logarithmic scale to highlight differences in isotherm slope. The design of stable adsorbents capable of selectively capturing dioxygen with a high reversible capacity is a crucial goal in functional materials development. Drawing inspiration from biological O 2 carriers, we demonstrate that coupling metal-based electron transfer with secondary coordination sphere effects in the metal–organic framework Co 2 (OH) 2 (bbta) (H 2 bbta = 1 H ,5 H -benzo(1,2- d: 4,5- d ′)bistriazole) leads to strong and reversible adsorption of O 2 . In particular, moderate-strength hydrogen bonding stabilizes a cobalt(III)-superoxo species formed upon O 2 adsorption. Notably, O 2 -binding in this material weakens as a function of loading, as a result of negative cooperativity arising from electronic effects within the extended framework lattice. This unprecedented behavior extends the tunable properties that can be used to design metal–organic frameworks for adsorption-based applications. Allosteric binding of substrates to biomolecules is effortlessly accomplished in nature, but engineering synthetic materials to display similarly responsive behavior remains an ongoing challenge. In addition to non-cooperative substrate binding (e.g., O 2 in myoglobin), biomolecules can exhibit cooperativity arising from structural changes that strengthen or weaken interactions with substrates. Positive cooperativity can lead to enhanced response to ligands under certain conditions (e.g., O 2 binding in hemoglobin), while negative cooperativity generates a weakened response to successive binding events and enables biomolecules to maintain molecule sensitivity over greater concentration ranges than observed for non-cooperative or positively cooperative proteins (e.g., insulin binding to the insulin receptor) [1] , [2] , [3] , [4] . The ability to reproduce similar performance in synthetic materials could be advantageous for a multitude of potential applications, including catalysis [5] , [6] , sensing [7] , and gas separations [8] , [9] . Metal–organic frameworks provide an intriguing platform for the design and study of cooperative adsorption, owing to their crystallinity, chemical versatility, and extended network structure that can readily propagate minor structural changes [10] , [11] . Indeed, some of us have recently shown that cooperative CO 2 uptake in alkyldiamine-appended M 2 (dobpdc) (M = Mg, Mn, Fe, Co, Ni, Zn; H 4 (dobpdc) = 4,4′-dioxidobiphenyl-3,3′-dicarboxylic acid) occurs as a result of the extended formation of ammonium carbamate chains down the framework pores [8] , while the propagation of an iron(II) spin transition upon CO binding gives rise to its cooperative adsorption in the frameworks Fe 2 Cl 2 (bbta) (H 2 bbta = 1 H ,5 H -benzo(1,2- d :4,5- d ′)bistriazole) and Fe 2 Cl 2 (btdd) (H 2 btdd = bis(1 H -1,2,3-triazolo[4,5- b ],[4′,5′- i ])dibenzo[1,4]dioxin) [9] . The adsorption behavior of these materials stands in stark contrast to the non-cooperative, Langmuir-type uptake that is typical of frameworks featuring isolated binding sites (Fig. 1 ). As a result, these cooperative adsorbents exhibit exceptionally high selectivities and capacities and can be regenerated with far lower energy costs than traditional adsorbents, rendering them of interest for industrial separation applications. Fig. 1: Illustration of adsorption isotherm variability with cooperativity. Isotherms of positively cooperative (red line), noncooperative (purple line), and negatively cooperative (blue line) systems exhibit significant differences in shape, due to the nature of the adsorbate-adsorbent interactions. In particular, negatively cooperative systems can reach half occupancy at significantly lower pressures than noncooperative and positively cooperative systems but generally require much higher pressures to reach saturation. The inset graph displays the low pressure regime (<0.2 bar) on a logarithmic scale to highlight differences in isotherm slope. Full size image The development of a metal–organic framework capable of cooperative O 2 adsorption could be advantageous for a number of applications in industry, including energy-efficient O 2 production [11] , [12] , O 2 storage [13] , [14] , [15] , and catalysis [16] , [17] . Iron- [18] , [19] , chromium- [20] , [21] , manganese- [22] , copper- [23] , and cobalt-based [24] , [25] frameworks have previously been shown to bind O 2 via reversible reduction upon metal coordination, but the poor chemical stability of many of these materials to O 2 limits their cyclable capacity under ambient conditions. In the search for improved, cooperative adsorbents for O 2 capture, the active sites of proteins such as hemoglobin, hemerythrin, and hemocyanin can serve as sources of inspiration. 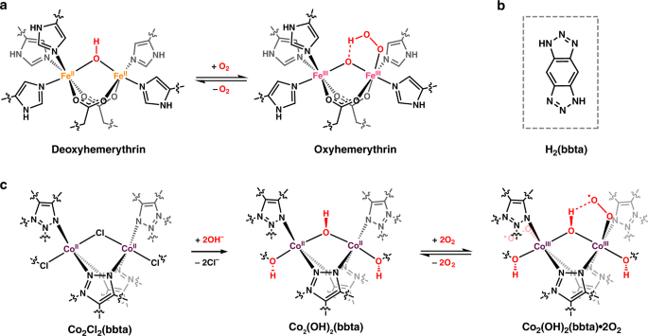Fig. 2: Hydrogen bond stabilization of dioxygen binding in hemerythrin. aIllustration of O2binding in the metalloprotein hemerythrin, which shows the critical role that the bridging hydroxo group of the active site plays in the stabilization of the resulting iron(III)-hydroperoxo species.bThe structure of the H2bbta ligand, 1H,5H-benzo(1,2-d:4,5-d′)bistriazole), used in this work.cIllustration of post-synthetic modification of Co2Cl2(bbta) by anion exchange with OH−(left) to form Co2(OH)2(bbta) (middle)33. The bridging hydroxo groups in this structure provide stabilization to bound O2(right) in a manner analogous to oxyhemerythrin. These sites feature reducing transition metal centers that bind O 2 via electron transfer to reversibly generate metal-superoxo or metal-peroxo species [26] , [27] , and crucially these species are often stabilized through directed hydrogen-bonding interactions [28] . For example, histidine residues in hemoglobin hydrogen bond to the iron-superoxo formed upon O 2 uptake [28] , [29] , while in hemerythrin a bridging hydroxo group transfers a proton to iron-bound dioxygen to form a hydroperoxo species (Fig. 2a ) [30] . These hydrogen bonding interactions are thought to play a key role in reversible O 2 binding in these proteins, and may also be advantageous for the development of metal–organic frameworks for selective and reversible O 2 capture. Here, we report the detailed characterization of O 2 adsorption in the frameworks Co 2 X 2 (bbta) (X − = Cl − , OH − ) [31] , [32] , [33] , [34] and show that Co 2 (OH) 2 (bbta) is able to capture O 2 with high affinity by leveraging both electron transfer and hydrogen bonding interactions (Fig. 2c ). Remarkably, as a result of the close metal contacts within Co 2 (OH) 2 (bbta), O 2 interacts more weakly with the cobalt(II) centers upon increased loading, providing the first clear example of an adsorbent material that exhibits negative cooperativity upon gas binding. Fig. 2: Hydrogen bond stabilization of dioxygen binding in hemerythrin. a Illustration of O 2 binding in the metalloprotein hemerythrin, which shows the critical role that the bridging hydroxo group of the active site plays in the stabilization of the resulting iron(III)-hydroperoxo species. b The structure of the H 2 bbta ligand, 1 H ,5 H -benzo(1,2- d: 4,5- d ′)bistriazole), used in this work. c Illustration of post-synthetic modification of Co 2 Cl 2 (bbta) by anion exchange with OH − (left) to form Co 2 (OH) 2 (bbta) (middle) [33] . The bridging hydroxo groups in this structure provide stabilization to bound O 2 (right) in a manner analogous to oxyhemerythrin. Full size image Design, synthesis, and gas adsorption properties In our search for a cooperative, O 2 -selective metal–organic framework, we initially investigated the known framework Co 2 Cl 2 (bbta), which features a high density of coordinatively-unsaturated cobalt(II) ions [31] , [32] , as well as basic nitrogen-donor ligands that should enhance the reducing potential of the metal centers [24] . However, we found that Co 2 Cl 2 (bbta) exhibits only a weak interaction with oxygen (Fig. 3a ), indicating that the ligand environment is not basic enough to facilitate metal-centered O 2 reduction, and we thus turned our attention to the recently reported derivative Co 2 (OH) 2 (bbta) (Fig. 2c ) [33] . Synthesis of this material following a significantly modified procedure (see the Supporting Methods) led to a crystalline compound with a Brunauer–Emmett–Teller surface area of 1470 m 2 g −1 (Supplementary Figs. 2 – 4 ). Fig. 3: Oxygen adsorption data. a Oxygen adsorption isotherms obtained at 195 K for Co 2 Cl 2 (bbta) (gold circles) and Co 2 (OH) 2 (bbta) (purple circles). b Oxygen adsorption isotherms obtained at 195, 213, and 223 K for Co 2 (OH) 2 (bbta) (maroon, red, and orange symbols respectively). Symbols represent data points and lines represent fits using a dual-site Langmuir model. The inset depicts the differential enthalpy of adsorption for O 2 adsorption in Co 2 (OH) 2 (bbta) (gray line, with error bars), determined using the Clausius–Clapeyron equation as described in the Methods. Source data are provided as a source data file. Full size image At 195 K, the O 2 adsorption isotherm for Co 2 (OH) 2 (bbta) exhibits a sharp rise at low pressures (Fig. 3a ), and the material achieves a capacity of ∼ 3 mmol g −1 (0.47 mmol O 2 per mmol Co) at just 25 mbar. At 1 bar, the capacity is 7.57 mmol g −1 (19.5 wt % or 1.17 mmol O 2 per mmol Co), significantly higher than that of Co 2 Cl 2 (bbta) under the same conditions (3.24 mmol g −1 , or 0.63 mmol O 2 per mmol Co) and higher than any other cobalt(II)-based framework studied for O 2 adsorption [24] , [25] . To quantify the strength of the metal–O 2 interactions in Co 2 (OH) 2 (bbta), we determined the differential enthalpy of O 2 adsorption (Δ h ads ) from the Clausius–Clapeyron equation, using parameters extracted from a dual-site Langmuir fit of adsorption isotherms collected at 195, 213, and 223 K (Fig. 3b and Methods). At low loadings, O 2 occupies a primary binding site with Δ h ads = −49 ± 2 kJ mol −1 , which is more than three times the differential enthalpy of O 2 adsorption in Co 2 Cl 2 (bbta), and with a saturation capacity of 2.46 ± 0.02 mmol g −1 (approximately 0.38 mmol O 2 per mmol Co; Fig. 3b ). Consistent with these results, density functional theory (DFT) calculations performed on various model systems indicate that Co 2 (OH) 2 (bbta) has a much higher affinity for O 2 than Co 2 Cl 2 (bbta) (Supplementary Tables 43 and 47 ). In tandem with the comparatively high adsorption site density in Co 2 (OH) 2 (bbta) per formula weight [24] , [25] , this large enthalpy of adsorption explains the high uptake capacity of the material. The primary binding site also exhibits a large differential entropy of adsorption (Δ s ads ) of 186 ± 7 J mol −1 K −1 , leading to a significant adsorption temperature dependence that accounts for the low uptake at 298 K (Fig. 3b ; Supplementary Figs. 6 and 15 ). With increasing loading, O 2 occupies a secondary binding site with Δ h ads = −18 ± 2 kJ mol −1 . Despite the high differential enthalpy observed at low loadings, O 2 adsorption was found to be fully reversible under all temperatures and pressures studied. Importantly, the capacity and differential enthalpy of O 2 adsorption in Co 2 (OH) 2 (bbta) are substantially greater than those values measured and determined for N 2 (Supplementary Figs. 10 , 11 , and 14 ). Ideal adsorbed solution theory [35] was used to calculate the O 2 /N 2 selectivities for a mixture containing 21% O 2 and 79% N 2 , representative of air (Supplementary Table 5 ). At 195 K, the calculated selectivity is 42, similar to that reported for the framework Co-BTTri (Co 3 [(Co 4 Cl) 3 (BTTri) 8 ] 2 ; H 3 BTTri = 1,3,5-tri(1 H -1,2,3-triazol-5-yl)benzene) under the same conditions (41) [24] , and this value decreases with increasing temperature to 14 at 223 K. These selectivities correspond, respectively, to 91% and 79% pure adsorbed O 2 on Co 2 (OH) 2 (bbta) under equilibrium conditions. 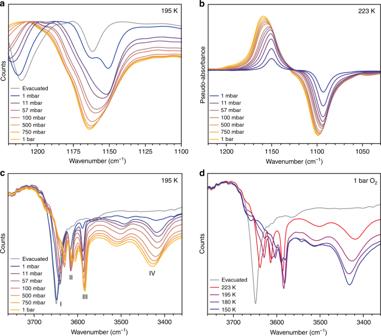Fig. 5: Spectroscopic data for evacuated and O2-dosed Co2(OH)2(bbta). aRaw DRIFTS data obtained at 195 K by dosing Co2(OH)2(bbta) with variable pressures of16O2.bDRIFTS spectra obtained at 223 K for Co2(OH)2(bbta) dosed with increasing pressures of16O2, subtracted from the spectra of Co2(OH)2(bbta) dosed with corresponding pressures of18O2. The ν(O–O) band of the adsorbed superoxo species appears as a positive peak for16O2and a negative peak for18O2.cRaw DRIFTS spectra obtained at 195 K for desolvated and16O2-dosed Co2(OH)2(bbta). The broad ν(OH) band from 3416–3427 cm−1(IV) is assigned to a cobalt(III)-hydroxo hydrogen bonded to the proximal oxygen atom of an adsorbed superoxo species. Sharper peaks (I–III) correspond to additional framework hydroxo groups, as indicated in Supplementary Fig.54.dRaw DRIFTS spectra obtained at 223 K for desolvated Co2(OH)2(bbta) and for Co2(OH)2(bbta) dosed with 1 bar of16O2obtained at 223, 195, 180, and 150 K. 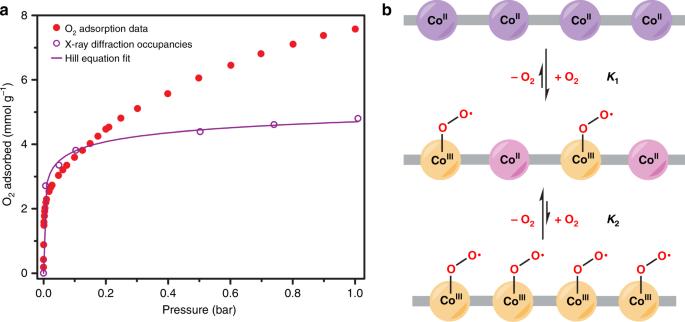Fig. 6: Negative cooperativity of O2binding. aOxygen adsorption isotherm obtained at 195 K for Co2(OH)2(bbta) (filled red circles) plotted alongside values obtained for superoxo occupancies under similar conditions with powder X-ray diffraction data, multiplied by the theoretical capacity of 6.45 mmol g−1(open purple circles). Modeling these occupancy values using the Hill equation resulted in excellent agreement (solid purple line; Supplementary Information Sections8). At low pressures, the projected capacity values from the diffraction occupancies are very slightly higher than the experimental adsorption capacities, which may be due to adsorption at defects (e.g., surface sites) that are not reflected in the occupancies. At higher pressures, the significant deviation of the gas adsorption from the projected occupancy capacities is due to physisorption within the pore. Source data are provided as a source data file.bSimplified illustration of a chain of cobalt centers in Co2(OH)2(bbta) running along the c-axis in the activated material (top), following oxidation to generate cobalt(III)-superoxo species (yellow spheres) and unreacted, less electron-rich cobalt(II) ions (pink spheres) (middle), and the fully oxidized cobalt(III)-superoxo chain (bottom). From analysis of the variable-temperature O2adsorption data, the equilibrium constant for partial O2loading (K1) is estimated to be much larger than the equilibrium constant to achieve 100% occupancy (K2). As a result, the partially oxidized material dominates under all conditions studied here. Notably, Co 2 (OH) 2 (bbta) also exhibits an O 2 working capacity of 1.5 mmol g −1 (4.6 wt %) upon lowering the pressure from 0.21 to 0.05 bar at 195 K, which is higher than the values reported for Co-BTTri and Fe 2 (dobdc) [24] . Together, these results suggest that Co 2 (OH) 2 (bbta) could potentially be useful for air separation in a vacuum-swing adsorption process. Structural, spectroscopic, and magnetic characterization The solid-state structure of Co 2 (OH) 2 (bbta) was determined from Rietveld refinement against neutron powder diffraction data collected on the desolvated material (obtained under vacuum at 6 K; see Fig. 4a ). The framework features hexagonal channels lined with rows of coordinatively-unsaturated cobalt(II) centers that are bridged by a combination of hydroxo and triazolate groups (Fig. 4b,c ). The Co–N bond lengths (2.066(17) and 2.102(4) Å) are within the range expected for nitrogen-donor ligands bound to high-spin cobalt(II) [36] . Analysis of in situ X-ray powder diffraction data for a sample of Co 2 (OH) 2 (bbta) dosed with increasing pressures of O 2 at 195 K revealed a gradual shift in the allowed reflections to higher angles, indicative of a unit cell contraction with increased O 2 loading (Supplementary Fig. 23 ). For example, dosing with 1 bar of O 2 resulted in an 8.6% decrease in the unit cell volume (Supplementary Tables 9 and 10 ) relative to the activated framework, concomitant with a decrease in the cobalt–ligand bond distances, from 2.072(6) to 1.956(5) Å ( d Co–OH ) and from 2.115(8)/2.007(13) Å to 1.932(10)/1.956(14) Å ( d Co–N ). Rietveld refinements against this variable-pressure data yielded structural models consistent with the presence of end-on cobalt(III)-superoxo species under all conditions (Fig. 4d ; ∠ Co–O–O = 119.9(4)°, 75(1)% occupancy) [26] . This metrical data is supported by values determined from periodic DFT calculations ( d O–O = 1.30 Å and and d Co–O = 1.87 Å for Co 2 (OH) 2 (bbta)·2O 2 ; see Supplementary Information Section 16 ). While there is evidence for physisorption of O 2 along the pore walls at high pressures, the superoxo site occupancy also grows with increasing pressure at 195 K, a change associated with an increasing unit cell volume contraction (Supplementary Fig. 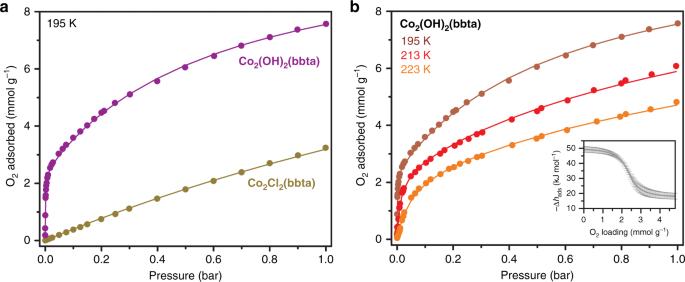25 ). Fig. Fig. 3: Oxygen adsorption data. aOxygen adsorption isotherms obtained at 195 K for Co2Cl2(bbta) (gold circles) and Co2(OH)2(bbta) (purple circles).bOxygen adsorption isotherms obtained at 195, 213, and 223 K for Co2(OH)2(bbta) (maroon, red, and orange symbols respectively). Symbols represent data points and lines represent fits using a dual-site Langmuir model. The inset depicts the differential enthalpy of adsorption for O2adsorption in Co2(OH)2(bbta) (gray line, with error bars), determined using the Clausius–Clapeyron equation as described in the Methods. Source data are provided as a source data file. 4: Structures of activated and O 2 -dosed Co 2 (OH) 2 (bbta). a – c Structures of activated Co 2 (OH) 2 (bbta) as determined by Rietveld refinement against neutron powder diffraction data obtained at 8 K, showing a the hexagonal framework channels with the view down the c axis, b a truncated view of the coordinatively-unsaturated metal centers lining the pores, and c a single coordinatively-unsaturated cobalt(II) center. d Structure of Co 2 (OH) 2 (bbta) dosed with 1 bar of O 2 , as determined from Rietveld refinement against powder X-ray diffraction data obtained at 195 K. Hydrogen atom positions could not be determined from the measurement. The 0.46 equivalents of O 2 found within the pores are not shown for clarity. e Structure of Co 2 (OH) 2 (bbta)(O 2 ) 1.74 ·(O 2 ) 0.17 determined from Rietveld refinement against neutron powder diffraction data of Co 2 (OH) 2 (bbta) dosed with 1 equivalent of O 2 per cobalt at 8 K. The 0.17 equivalents of O 2 found within the pores are not shown for clarity. In b , c , and e , only one orientation is shown for the half-occupancy hydrogen atom of the hydroxo group. Slight deviations in the bond distances derived from the neutron and X-ray diffraction data are likely a result of differences in experimental conditions, as well as the improved scattering of the O atoms in neutron diffraction. Purple, red, blue, gray, and white spheres represent Co, O, N, C, and H atoms, respectively. Full size image In situ diffuse reflectance infrared Fourier transform spectroscopy (DRIFTS) was used to further investigate the nature of the Co–O 2 interaction upon O 2 adsorption in Co 2 (OH) 2 (bbta). Dosing the framework with 1 mbar of 16 O 2 at 195 K afforded a new peak in the spectrum at 1151 cm −1 (Fig. 5a ), which can be assigned to the ν (O–O) band of a superoxide (O 2 − ) species bound end-on to cobalt(III) (1200–1100 cm −1 ) [26] . This peak shifts by 57 cm −1 to 1094 cm −1 when the material is dosed with 1 mbar of 18 O 2 (Fig. 5b ), close to the isomer shift of 69.1 cm −1 predicted from the single harmonic oscillator model for O 2 (Supplementary Figs. 49 and 50 ) [37] . Additionally, the superoxo overtone shifts from 2288 to 2182 cm −1 (Supplementary Fig. 46 ). Consistent with our experimental results, Kohn-Sham DFT calculations predicted the formation of superoxo species exhibiting an O–O stretching frequency shift of ∼ 400 cm –1 with respect to the gas phase value (Supplementary Information Section 17 ). As observed in the isotherm data (Supplementary Fig. 5 ), O 2 adsorption was found to be fully reversible upon evacuation of the sample at 195 K or heating at ambient pressure above 250 K. Fig. 5: Spectroscopic data for evacuated and O 2 -dosed Co 2 (OH) 2 (bbta). a Raw DRIFTS data obtained at 195 K by dosing Co 2 (OH) 2 (bbta) with variable pressures of 16 O 2 . b DRIFTS spectra obtained at 223 K for Co 2 (OH) 2 (bbta) dosed with increasing pressures of 16 O 2 , subtracted from the spectra of Co 2 (OH) 2 (bbta) dosed with corresponding pressures of 18 O 2 . The ν(O–O) band of the adsorbed superoxo species appears as a positive peak for 16 O 2 and a negative peak for 18 O 2 . c Raw DRIFTS spectra obtained at 195 K for desolvated and 16 O 2 -dosed Co 2 (OH) 2 (bbta). The broad ν(OH) band from 3416–3427 cm −1 (IV) is assigned to a cobalt(III)-hydroxo hydrogen bonded to the proximal oxygen atom of an adsorbed superoxo species. Sharper peaks (I–III) correspond to additional framework hydroxo groups, as indicated in Supplementary Fig. 54 . d Raw DRIFTS spectra obtained at 223 K for desolvated Co 2 (OH) 2 (bbta) and for Co 2 (OH) 2 (bbta) dosed with 1 bar of 16 O 2 obtained at 223, 195, 180, and 150 K. Full size image Variable-temperature d.c. magnetic susceptibility data were collected on samples of Co 2 (OH) 2 (bbta) before and after exposure to O 2 ( H d.c. = 0.1 T). At 300 K, the molar magnetic susceptibility times temperature ( χ M T ) for the desolvated material is 4.84 emu K mol −1 . This value is larger than that predicted for two high-spin S = 3/2 cobalt(II) centers (3.75 emu K mol −1 ), likely due to contributions from orbital angular momentum (Supplementary Fig. 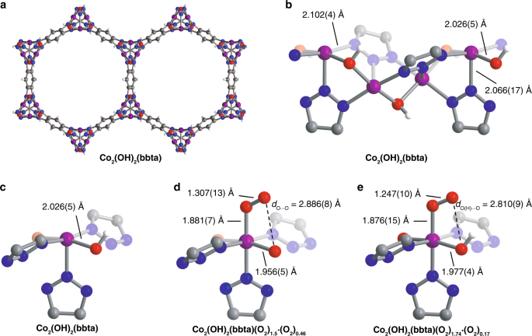63 ). With decreasing temperature, χ M T decreases gradually, reaching 0.274 emu K mol −1 at 2 K. Interestingly, the material also exhibits a negative Curie-Weiss constant ( θ = −81.0 K; Supplementary Fig. Fig. 4: Structures of activated and O2-dosed Co2(OH)2(bbta). a–cStructures of activated Co2(OH)2(bbta) as determined by Rietveld refinement against neutron powder diffraction data obtained at 8 K, showingathe hexagonal framework channels with the view down the c axis,ba truncated view of the coordinatively-unsaturated metal centers lining the pores, andca single coordinatively-unsaturated cobalt(II) center.dStructure of Co2(OH)2(bbta) dosed with 1 bar of O2, as determined from Rietveld refinement against powder X-ray diffraction data obtained at 195 K. Hydrogen atom positions could not be determined from the measurement. The 0.46 equivalents of O2found within the pores are not shown for clarity.eStructure of Co2(OH)2(bbta)(O2)1.74·(O2)0.17determined from Rietveld refinement against neutron powder diffraction data of Co2(OH)2(bbta) dosed with 1 equivalent of O2per cobalt at 8 K. The 0.17 equivalents of O2found within the pores are not shown for clarity. Inb,c, ande, only one orientation is shown for the half-occupancy hydrogen atom of the hydroxo group. Slight deviations in the bond distances derived from the neutron and X-ray diffraction data are likely a result of differences in experimental conditions, as well as the improved scattering of the O atoms in neutron diffraction. Purple, red, blue, gray, and white spheres represent Co, O, N, C, and H atoms, respectively. 65 ) and multireference methods and Kohn-Sham DFT calculations on di- and tetracobalt cluster models of Co 2 (OH) 2 (bbta), predict that an antiferromagnetic ground state for the high-spin cobalt ions is slightly more stable (4 kJ mol −1 , Supplementary Table 41 ) than a ferromagnetic ground state (Supplementary Information Section 15 ). The χ M T curves for Co 2 (OH) 2 (bbta)·O 2 and Co 2 (OH) 2 (bbta)·2O 2 exhibit a clear sigmoidal shape (Supplementary Fig. 64 ), which is reminiscent of that observed for spin crossover materials [38] and indicates temperature-dependent framework oxidation. At 100 K, the χ M T value for Co 2 (OH) 2 (bbta)·2O 2 (1 O 2 per Co) is 2.28 emu K mol −1 , very close to the spin-only value of 2.25 emu K mol −1 expected for one cobalt(III) ion ( S = 0), one cobalt(II) ion ( S = 3/2), and one superoxide ( S = 1/2), in the absence of magnetic exchange. DFT calculations at the PBE0-D3 level suggest that the spin density of cobalt changes from 2.67 to 0.07 upon O 2 adsorption, while the spin density of O 2 changes from 1.8 to 0.79 (Supplementary Table 43 ). Together with the diffraction and DRIFTS data, these results indicate that adsorbed O 2 is reduced by cobalt(II), yielding a superoxo-bound cobalt(III) species. Hydrogen bond stabilization of the superoxo species In the X-ray powder diffraction derived structure of Co 2 (OH) 2 (bbta) dosed with 1 bar of O 2 at 195 K, the terminal superoxo oxygen and the hydroxo oxygen are separated by only 2.886(8) Å, within the range for a moderate-strength O(H) · · · O hydrogen bonding interaction (Fig. 4c ) [39] . Refinement against neutron powder diffraction data collected on a sample dosed with 1 equiv. of O 2 per Co and cooled to 8 K notably revealed a hydrogen atom interacting with the terminal superoxo oxygen ( ∠ O–H · · · O = 108°, Fig. 4d ) [39] , [40] . Exclusion of this hydrogen atom from the refinement resulted in significantly worse goodness-of-fit parameters and a clear negative peak in the Fourier difference map (Supplementary Figs. 38 and 39 ). Notably, such a secondary coordination sphere effect upon O 2 -binding has not previously been observed in a metal–organic framework [41] , [42] , [43] , [44] . The presence of hydrogen bonding is supported by a comparison of the infrared spectra for desolvated and O 2 -dosed Co 2 (OH) 2 (bbta) (Fig. 5c,d ). A single ν (OH) band is present at 3648 cm −1 for the desolvated material (I, Fig. 4c , gray curve), while dosing with 1 mbar of O 2 leads to additional sharp bands at 3614 and 3586 cm −1 (II and III) and a broad band at ∼ 3420 cm −1 (IV). These three peaks redshift with increasing O 2 pressure up to 1 bar, and band III dominates at high pressures. The sharp features are assigned to –OH moieties that are not participating in hydrogen bonding but are affected by the redox changes of adjacent cobalt centers upon O 2 binding (Supplementary Fig. 54 ). Peak IV redshifts by >200 cm −1 relative to other ν (OH) resonances observed upon oxidation, and its energy is consistent with those reported for ν (OH) bands associated with O(H) · · · O interactions between 2.8 and 2.9 Å [40] . Thus, we assign this feature to an –OH adduct hydrogen bonding with a metal-bound superoxo. At higher O 2 occupancies (Fig. 4c ) or lower temperatures (Fig. 4d ), the broad band dominates and the sharp features at ∼ 3610 and ∼ 3580 cm −1 diminish. This trend is expected as O 2 loading increases and free –OH groups increasingly become engaged in hydrogen bonding. Interestingly, we do not observe full O 2 occupancy under any of the conditions measured here. Computed infrared spectra of the hydrogen-bonded cobalt(III)-superoxo in Co 2 (OH) 2 (bbta) successfully simulate the multiplicity of hydroxo peaks observed at low pressures (Supplementary Table 47 and Supplementary Fig. 87 ). Calculations examining three possible –OH group geometries indicate that the formation of a hydrogen bond to the cobalt(III)-superoxo lowers the O 2 adsorption energy by more than 20 kJ mol −1 (Supplementary Table 43 ). Significantly, this value is similar in magnitude to the calculated decrease in O 2 binding energy upon changing the framework from Co 2 Cl 2 (bbta) to Co 2 (OH) 2 (bbta) ( ∼ 30 kJ mol −1 ). Stabilization afforded by hydrogen bonding thus appears to be a critical factor leading to the high differential enthalpy of O 2 adsorption in Co 2 (OH) 2 (bbta). This interaction likely also facilitates stable, reversible O 2 binding, despite the strong cobalt(II)–O 2 interaction. Negative cooperativity of O 2 binding Adsorbate binding at coordinatively unsaturated metal sites is typically much stronger than physisorptive interactions [45] , [46] . However, in the case of Co 2 (OH) 2 (bbta), the O 2 occupancy determined from X-ray powder diffraction data at 195 K (75(1)%) is much greater than the saturation capacity of the strong site determined through the dual-site Langmuir model (2.46 ± 0.02 mmol g −1 , 38% occupancy). Additionally, our analysis of the variable-pressure DRIFTS spectra (Fig. 5a,b ) revealed an increase in integrated area that is greater than predicted for the strong binding site, based on analysis of adsorption data (Fig. 57) [47] . These results indicate that the Langmuir model does not accurately describe the O 2 binding to cobalt at all pressures. Significant IR peak asymmetry at higher loadings could be modeled as two Lorentzian peaks from 1149–1152 cm −1 and 1164–1167 cm −1 , with the higher energy band dominating at higher loadings (Supplementary Figs. 58 – 62 ). The same asymmetry is also clearly visible in spectra collected using 18 O 2 , confirming that it originates from changes in the bound superoxo species (Fig. 5b ). The shift of the band to higher energies further suggests a greater amount of electron transfer from the cobalt to adsorbed O 2 at lower pressures, resulting in a weaker O–O bond. Based on these data, we hypothesize that isolated cobalt(III)-superoxo species dominate at lower pressures, while at higher pressures an increase in the number of adjacent cobalt(III)-superoxo neighbors reduces the driving force for subsequent O 2 binding and reduction. Together with the adsorption and in situ diffraction data, these findings indicate that the interaction of O 2 with Co 2 (OH) 2 (bbta) changes drastically as a function of O 2 pressure at 195 K, resulting in incomplete occupation of the open metal sites, even at 1 bar. This attenuated affinity at higher pressures can be attributed to structural and electronic changes that disfavor further superoxo formation following each O 2 binding event, and is remarkably reminiscent of negative cooperativity in biological systems [2] , [3] , [48] . In particular, the initial binding of an O 2 molecule to a cobalt(II) center creates a comparatively electron-poor cobalt(III) center. Ligand-sharing cobalt(II) centers consequently become less electron donating, and higher pressures of O 2 are required to facilitate O 2 adsorption via electron transfer (Fig. 6 ). Computations further suggest that the reduced availability of hydroxo groups for hydrogen bonding may decrease the O 2 binding energy at high coverage (Supplementary Information Sections 16 and 17 ). Fig. 6: Negative cooperativity of O 2 binding. a Oxygen adsorption isotherm obtained at 195 K for Co 2 (OH) 2 (bbta) (filled red circles) plotted alongside values obtained for superoxo occupancies under similar conditions with powder X-ray diffraction data, multiplied by the theoretical capacity of 6.45 mmol g −1 (open purple circles). Modeling these occupancy values using the Hill equation resulted in excellent agreement (solid purple line; Supplementary Information Sections 8 ). At low pressures, the projected capacity values from the diffraction occupancies are very slightly higher than the experimental adsorption capacities, which may be due to adsorption at defects (e.g., surface sites) that are not reflected in the occupancies. At higher pressures, the significant deviation of the gas adsorption from the projected occupancy capacities is due to physisorption within the pore. Source data are provided as a source data file. b Simplified illustration of a chain of cobalt centers in Co 2 (OH) 2 (bbta) running along the c-axis in the activated material (top), following oxidation to generate cobalt(III)-superoxo species (yellow spheres) and unreacted, less electron-rich cobalt(II) ions (pink spheres) (middle), and the fully oxidized cobalt(III)-superoxo chain (bottom). From analysis of the variable-temperature O 2 adsorption data, the equilibrium constant for partial O 2 loading ( K 1 ) is estimated to be much larger than the equilibrium constant to achieve 100% occupancy ( K 2 ). As a result, the partially oxidized material dominates under all conditions studied here. Full size image X-ray powder diffraction occupancy results were modeled using the Hill equation, yielding a Hill coefficient of n = 0.262, consistent with a negatively cooperative adsorption mechanism (Fig. 6 and Supplementary Information Sections 8 ; generally n « 1 for negatively cooperative systems) [49] . The absence of saturation in our material, defined here as the adsorption of less than one O 2 per cobalt center, was further modeled using a Markov chain simulation (Methods and Supplementary Information Sections 14 ). In this simplified scenario, addition of O 2 to a chain of cobalt atoms is disfavored if the gas is already adsorbed at an adjacent site. With this model, the simulated occupancy of cobalt approaches 42%, in agreement with the saturation capacity of the strong binding site at low pressures ( ∼ 38%). Thus, negative cooperativity between the open cobalt sites appears integral to the adsorption behavior of O 2 in Co 2 (OH) 2 (bbta). Negatively cooperative systems display a weakened response to increasing equivalents of ligand, enabling them to maintain a sensitivity to substrate concentration through much greater ranges than experienced in non-cooperative or positively cooperative systems [1] , [2] , [3] . As a result, an adsorbent exhibiting negatively cooperative guest binding would continue to adsorb even at high pressures, leading to significant working capacities over a large range of conditions, as is demonstrated here for Co 2 (OH) 2 (bbta). The foregoing results show that the framework Co 2 (OH) 2 (bbta) adsorbs O 2 at low temperatures via reversible reduction to form cobalt(III)-superoxo species. At low pressures, Co 2 (OH) 2 (bbta) exhibits higher capacities and stronger binding of O 2 than any other reported cobalt(II) metal–organic framework and may therefore be a promising candidate for O 2 -selective air separations. Crucially, the highly basic hydroxo ligands in this material increase the reducing potential of the cobalt(II) sites and also engage in secondary-sphere hydrogen bonding interactions with bound superoxo groups, affording stabilization analogous to that observed in biological O 2 carriers and biomimetic O 2 -binding molecules [28] , [29] , [41] , [50] , [51] , [52] . Unexpectedly, this allosteric behavior also leads to a negative cooperativity for O 2 binding, which is unprecedented in an extended framework material, though one previous example involving a molecular complex within a zeolite was found to display a Hill coefficient of 0.51 [53] . This behavior can be contrasted to the positive cooperativity observed of CO binding in the isostructural framework Fe 2 Cl 2 (bbta) [9] , demonstrating how precise atomic control in the synthesis and modification of these materials can yield complex and emergent biomimetic properties. General considerations The ligand H 2 (bbta) was synthesized according to a previously published procedure [33] . All other reagents were obtained from commercial vendors and used as received. Ultra-high purity grade (99.999% purity, Praxair) He, N 2 , and O 2 were used for all adsorption, spectroscopy, magnetometry, neutron, and X-ray diffraction measurements. After desolvation, all metal–organic framework samples were stored and handled under an N 2 atmosphere using standard glove box techniques. Elemental analyses (C, H, and N) were obtained from the Microanalytical Laboratory at the University of California, Berkeley; Co and Cl analyses were obtained from Galbraith Laboratories, Inc. Certain commercial equipment, instruments, or materials are identified in this paper to foster understanding. Such identification does not imply recommendation or endorsement by the National Institute of Standards and Technology, nor does it imply that the materials or equipment identified are necessarily the best available for the purpose. Synthesis of Co 2 (OH) 2 (bbta) Co 2 Cl 2 (bbta) was synthesized and desolvated according to a previously reported procedure [33] . Desolvated Co 2 Cl 2 (bbta) (100.0 mg, 0.3226 mmol) was soaked in a solution of 1 M (M = mol L −1 ) aqueous ammonia (100 mL) at room temperature for 24 h. The suspension was filtered and soaked in aqueous ammonia two more times before being filtered and soaked in water at room temperature for 3 days. The water was replaced every 24 h until the supernatant pH was no longer basic, as tested by pH paper. The suspension was then filtered, rinsed with methanol, and the resulting yellow-orange powder was heated at 160 °C under vacuum for 12 h. Anal. Calcd for Co 2 O 2 C 6 N 6 H 4 (%): C, 23.25; H, 1.30; N, 27.11; Co, 27.03*; Cl, 0; Cl/Co = 0. Found (%): C, 24.08; H, 1.00; N, 27.38; Co, 26.6(4); Cl, <0.01; Cl/Co = < 0.00037. *For Co 2 (OH) 2 (bbta)·7(H 2 O) Gas adsorption Gas adsorption isotherms for pressures in the range 0–1.2 bar were measured by a volumetric method using a Micromeritics ASAP 2020 instrument. A typical sample of ca. 50 mg of material was transferred to a pre-weighed analysis tube, which was capped with a transeal and evacuated by heating under dynamic vacuum until an outgas rate of less than 2.6 μbar min −1 was achieved. The evacuated analysis tube containing the degassed sample was then carefully transferred to an electronic balance and weighed again to determine the mass of sample. The tube was then transferred back to the analysis port of the gas adsorption instrument. The outgas rate was again confirmed to be less than 2.6 μbar min −1 . For all isotherms, warm and cold free space correction measurements were performed using ultra-high purity He gas; N 2 isotherms at 77 K were measured in liquid nitrogen baths, using UHP-grade gas sources and all room temperature measurements were measured with an insulated water bath. Oil-free vacuum pumps and oil-free pressure regulators were used for all measurements to prevent contamination of the samples during the evacuation process or of the feed gases during the isotherm measurements. Langmuir surface areas were determined from N 2 adsorption data at 77 K using Micromeritics software. Gas adsorption isotherms at 195 K were measured using baths with dry ice and isopropanol, and temperatures between −70 and −40 °C were measured using a Julabo immersion cooler with silicone-based Julabo thermal bath fluid. In all measurements, equilibration was determined by a change of less than 0.010% over a minute in the pressure over the sample, which typically involved each measurement point taking half an hour or longer. Adsorption isotherm fitting Adsorption isotherms for the uptake of O 2 in Co 2 (OH) 2 (bbta) at 195, 213, and 223 K were adequately fit with a dual-site Langmuir equation (Eq. 1 ), where n is the amount adsorbed in mmol g −1 , n sat,i is the saturation capacity in mmol g −1 , b i is the Langmuir parameter in bar −1 , and P is the pressure in bar. n = n_sat,1b_1P/1 + b_1P + n_sat,2b_2P/1 + b_2P
 (1) 
    b_i = e^S_i/Re^ - E_i · 1000/RT
 (2) The Langmuir parameter can further be expressed using Eq. 2 , where S i is the site-specific integral entropy of adsorption in J mol −1 K −1 , E i is the site-specific differential enthalpy of adsorption in kJ mol −1 , R is the gas constant in J mol −1 K −1 , and T is the temperature in K. The isotherms were fit independently for each temperature. However, it should be noted that the saturation capacities, n sat,i , were fixed to the values determined from a simultaneous fit to all temperatures. The error for these values was determined using the program Origin and are determined to be 2.46 ± 0.02 and 8.3 ± 0.1 mmol g −1 for n sat,1 and n sat,2 , respectively. Differential enthalpy of adsorption calculations Using the dual-site and single-site Langmuir fits, the differential enthalpy of adsorption, Δ h ads , can be calculated as a function of the total amount of gas adsorbed, n , by using the Clausius−Clapeyron equation (Eq. 3 ), where R is the gas constant in J mol −1 K −1 , T is the temperature in K, n is the total amount adsorbed in mmol g −1 , and P is the pressure in bar. Δh_ads = - RT^2( ∂ln P/∂ T)_n
 (3) The Langmuir fits for O 2 and N 2 adsorption in Co 2 (OH) 2 (bbta) and Co 2 Cl 2 (bbta) were used to obtain the exact pressures that correspond to specific loadings at 195, 213, and 223 K with Mathematica 11.0. This was done at loading intervals of 0.05 mmol g −1 . At each loading, the slope of the best-fit line to ln( P ) versus 1/ T was calculated in order to obtain the differential enthalpy of adsorption. The y-intercepts of these linear trendlines are equal to −Δ s ads R −1 at each loading (with p 0 = 1 bar), and thus were used to determine the corresponding differential entropies of adsorption. The results are shown in Supplementary Fig. 14 and reported in Supplementary Tables 1 – 4 . To corroborate the use of the dual-site Langmuir fit for O 2 adsorption on Co 2 (OH) 2 (bbta), additional calculations were performed by fitting the O 2 isotherms independently by spline interpolation and utilizing those fits to determine the differential enthalpy of adsorption, as described above. The differential enthalpy of adsorption obtained through this method is similar within error to the values calculated using the dual-site Langmuir model, providing validation for interpreting the adsorption data with a dual-site Langmuir model (Supplementary Fig. 16 ). Ideal adsorbed solution theory and vacuum swing adsorption calculations Ideal adsorbed solution theory (IAST) [35] was used to predict mixed gas behavior (specifically, 0.21 bar O 2 and 0.79 bar N 2 ) from single-component O 2 and N 2 adsorption isotherms. IAST selectivities as a function of temperature were calculated using the Langmuir fits for O 2 and N 2 in Co 2 (OH) 2 (bbta) and listed in Supplementary Table 5 . The selectivity factor, S , is defined according to Eq. 4 , where n i is the amount adsorbed for each component as determined from IAST and x i is the mole fraction of each component in the gas phase at equilibrium. S = n_O_2/n_N_2/x_O_2/x_N_2
 (4) Vacuum swing adsorption capacities were determined by extrapolating the exact capacity of adsorbed O 2 on Co 2 (OH) 2 (bbta) at 0.05 and 0.21 bar O 2 pressure at 195 K, by using the Langmuir adsorption fits determined as described above (3.009 and 4.507 mmol g −1 respectively). The difference in these values leads to a working capacity of 1.498 mmol g −1 , higher values than seen in either Co-BTTri or Fe 2 (dobdc) [24] . X-ray powder diffraction Powder X-ray diffraction data for Co 2 Cl 2 (bbta) and Co 2 (OH) 2 (bbta) were collected on Beamline 17-BM-B at the Advanced Photon Source at Argonne National Laboratory. A sample of the fully desolvated framework ( ∼ 2 mg) was loaded into a 1.0 mm borosilicate capillary inside a N 2 -atmosphere glovebox, before being attached to a custom-designed valved gas-dosing cell and transferred to the goniometer head. Adsorbed N 2 was removed by evacuating in situ using a turbomolecular pump. Once diffraction patterns were obtained for the evacuated framework, the samples were dosed with O 2 (5 to 1000 mbar). Diffraction data were collected after allowing the samples to equilibrate for at least 30 min after each dose, as confirmed by a constant pressure readout and consistent diffraction patterns. An Oxford Systems Cryostream 800 was used to change the temperature between 100 and 298 K. All X-ray wavelengths were between 0.451 and 0.453 Å, and are specified for each experiment. Diffracted intensity was recorded by a PerkinElmer a-Si flat panel detector. In the case of Co 2 Cl 2 (bbta), the sample was dosed with 27 mbar of O 2 at 298 K and then slowly cooled to 110 K (2 K/min), while monitoring powder X-ray diffraction patterns during the temperature changes. X-ray powder diffraction analysis Precise unit cell parameters of evacuated Co 2 Cl 2 (bbta), O 2 -dosed Co 2 Cl 2 (bbta), evacuated Co 2 (OH) 2 (bbta), and O 2 -dosed Co 2 (OH) 2 (bbta) were obtained by structureless Pawley refinement, as implemented in TOPAS-Academic 4.1, and all were consistent with a hexagonal lattice, similar to those observed for Fe 2 Cl 2 (bbta) and other M 2 X 2 (bbta) frameworks [9] , [32] , [33] , [54] . The backgrounds of the patterns were modeled with Chebyshev polynomial functions that were used, along with the correct unit cell parameters, sample displacement and profile parameters, in the subsequent Rietveld refinements. Peak shapes were described with the fundamental parameters approach. The structural model for evacuated Fe 2 Cl 2 (bbta) was first used as a starting point for evacuated Co 2 Cl 2 (bbta) [9] . The positions and thermal displacement parameters of the cobalt and chloride atoms were freely refined, and the carbon and nitrogen atoms of the bbta 2− ligand were refined with soft constraints. A single refined thermal displacement parameter was assigned to all atoms of the bbta 2− ligand. Consistent with previous work as well as the needle-like crystal habit observed in the SEM images of Co 2 Cl 2 (bbta) (Supplementary Fig. 45 ), a single March-Dollase correction along the (0 0 1) direction provided an improvement in the goodness-of-fit parameters ( R wp improved by ∼ 1.3%). The Fourier difference map showed little evidence for electron density over the framework metal centers, indicating that the material was fully desolvated prior to the gas dosing experiments. The Rietveld refinement using O 2 -dosed Co 2 Cl 2 (bbta) data obtained at 110 K was approached by examining the influence of O 2 -dosing on the diffraction pattern of the parent framework. Only a slight unit cell contraction was observed at this temperature (<0.9%), with some slight intensity changes being the chief difference between the two patterns. The Fourier difference map showed evidence for O 2 adsorbed within the pores, and a species was modeled along the locations indicated by the map and then allowed to freely refine. Upon this refinement, the closest distance of O 2 from the cobalt ions is ∼ 2.7 Å, with few changes observed in the coordination environment of the cobalt ions otherwise. This distance suggests a weak interaction, consistent with the small differential enthalpy of adsorption of O 2 measured for this framework. As with the desolvated sample, a single March-Dollase correction applied along the (0 0 1) direction provided an improvement in the goodness-of-fit parameters ( R wp improved by 1.06%). The obtained structural model of desolvated Co 2 Cl 2 (bbta) was used as the starting point for the Rietveld refinement using the diffraction pattern of evacuated Co 2 (OH) 2 (bbta). The hydroxo oxygen atom and cobalt atom were freely refined, and the ligand atom positions were refined within soft restraints. A single refined thermal displacement parameter was assigned to all atoms of the bbta 2− ligand. In the course of the refinement, it should be noted that the combination of the special positions of the Co and O atoms and the shorter Co–O bond length ( ∼ 2.1 Å in comparison to the ∼ 2.4 Å Co–Cl bond distances observed in Co 2 Cl 2 (bbta)) cause the O–Co–O angle to approach 170°, rather than 180° as observed in Co 2 Cl 2 (bbta). As a result, the coordination environment of the cobalt centers deviates slightly from an ideal square pyramidal geometry. However, this geometry is also observed in the Rietveld refinements performed using the neutron powder diffraction data, and is not chemically unreasonable, particularly if some strain is imposed by the crystallographic lattice. The O–Co–O angle also appears to play a role in the unit cell volume of Co 2 (OH) 2 (bbta) being slightly bigger than that of Co 2 Cl 2 (bbta), despite Cl − having a larger ionic radius than OH − . As with Co 2 Cl 2 (bbta), single March-Dollase correction was applied along the (0 0 1) direction and provided a slight improvement in the goodness-of-fit parameters ( R wp improved by 0.3%), consistent with the needle-like crystal habit observed in the SEM images of Co 2 (OH) 2 (bbta). Additionally, there was little to no observable electron density over the metal center, indicating complete desolvation prior to the gas dosing experiments on the same sample. The structural model for the evacuated sample was used as the starting point for the determination of the structural models for Co 2 (OH) 2 (bbta) dosed with increasing pressures of O 2 (0.0067–1.01 bar). Upon gas dosing, significant unit cell contractions were observed (4427(3) Å 3 to 4047.4(5) Å 3 ), necessitating care in the refinement of the structural models from the evacuated material, as the starting point was quite far off. Soft constraints on the bbta 2− ligand bond lengths and angles were employed, and the cobalt and hydroxo oxygen atoms were refined within constraints. After the framework structure was approximately determined, a Fourier difference map was used to examine adsorbed species within the pores. From this map, a bent shape of unmodeled electron density could be distinguished above the metal centers of the framework, reminiscent of a disordered bent end-on superoxo species. When oxygen atoms were assigned to be within this unmodeled density and then freely refined, one atom appeared to be directly above the cobalt ion on the two-fold axis that runs through the metal center. The second atom, which refined to a position ∼ 1.3 Å away from the first, refined to a general position with approximately 0.5 occupancy of the first atom in a position close to the hydroxo oxygen atom ( ∼ 2.7–2.9 Å). At low pressures of O 2 , the species over the metal centers appeared to be the only significant adsorbed species. At higher dosed pressures of O 2 , additional electron density could be resolved in the pores. Specifically, a position in between the superoxo species and over the ligand appeared to be a preferred location for a physisorbed oxygen. However, this position appears to be highly disordered under the measured conditions, in contrast to structural models obtained from the powder neutron diffraction data described below. As with desolvated Co 2 (OH) 2 (bbta), a single March-Dollase correction applied along the (0 0 1) direction provided an improvement in the goodness-of-fit parameters ( R wp improved by 0.4%). In all structural models, hydrogen atoms were added to the benzene ring of bbta 2− ligand to yield a C–H distance of 1.09 Å. During the final refinement, all parameters were freely refined. The result of all Rietveld refinements using data collected on Co 2 Cl 2 (bbta) are reported in Supplementary Figs. 21 and 22 , and the parameters are listed in Supplementary Tables 6 – 8 . The result of all Rietveld refinements using powder X-ray diffraction data collected on the Co 2 (OH) 2 (bbta) framework are reported in Supplementary Tables 10 – 12 , and the refinements are shown in Supplementary Figs. 26 – 35 . We also collected powder X-ray diffraction data for desolvated Co 2 (OH) 2 (bbta) prepared according to a previously published procedure, via washing of Co 2 Cl 2 (bbta) with aqueous KOH [1] . The sample was washed as previously described, before being fully desolvated (activation conditions: 100 °C for 24 h) and packed into a 1.0 mm borosilicate capillary inside a nitrogen glovebox that was flame-sealed. The sample was then measured at Beamline 12.2.2 at the Advanced Light Source of Lawrence Berkeley National Laboratory under an average wavelength of 0.4948 Å at room temperature (see Supplementary Fig. 19 ). The diffraction data confirms that in our hands, the known preparation resulted in synthesis of a significant amount of Co(OH) 2 alongside Co 2 (OH) 2 (bbta), in contrast to the preparation using aqueous ammonia washes. Neutron powder diffraction collection and analysis Powder neutron diffraction data were collected on 0.485 g of desolvated Co 2 (OH) 2 (bbta), loaded into a vanadium sample can in a helium glovebox. The sample can was sealed with an indium o-ring onto a copper heating block containing a valved outlet for gas loading. Data were collected at the high-resolution powder diffractometer, BT1, at the National Institute of Standards and Technology Center for Neutron Research, utilizing a Ge(311) monochromator with an in-pile 60’ collimator, corresponding to a neutron wavelength of 2.0772 Å. After mounting the sample to a bottom-loaded closed cycle refrigerator, the sample was cooled to 6 K for measurement, and subsequent measurements were collected at 150 and 300 K (Supplementary Fig. 33 ). For gas loading, the sample was dosed with ∼ 1 equiv. of O 2 per cobalt at 100 K, with adsorption verified barometrically prior to cooling to 8 K to avoid condensation. Measurements were then conducted at 8, 150, and 300 K, then at 150 and 8 K. Diffraction patterns for initial and final 8 and 150 K data sets were virtually identical (Supplementary Fig. 35 ). Powder neutron diffraction data was analyzed using GSAS [55] . Initially, Le Bail refinements were conducted to determine the profile parameters, after which Rietveld refinements were conducted. Bond restraints were initially placed on all bonds, based on chemical information. Final refinements only included bond restraints on the phenyl ring, with minimal impact. Occupancies that refined within unity (the atoms of bbta 2− linker, the Co atom, and the O atom of the OH − groups), were fixed. The thermal parameters of the bbta 2− linker were constrained to the same value. During the final refinements, the profile parameters, all atomic positions, and the occupancies were all refined, for both the gas-dosed and bare structures. The parameters are listed in Supplementary Tables 13 – 16 , and the refinements are shown in Supplementary Figs. 34 , 36 , and 37 . To confirm the position of the hydrogen atom of the hydroxo groups, a Rietveld refinement was performed where the hydroxo hydrogen atom was omitted from the structure, while keeping all other aspects of the refinement constant, and a Fourier difference map ( F obs – F calc ) was calculated from the refinement. The diminished goodness-of-fit parameters and the clear presence of well-localized atoms in the negative component of the different map (Supplementary Figs. 38 and 39 ) confirm the assignment of the hydrogen atom and its ability to hydrogen bond to the superoxo oxygen atom(d H···O = 2.35(2) Å). Infrared spectroscopy Infrared spectra were collected using a Bruker Vertex 70 spectrometer equipped with a glowbar source, KBr beamsplitter, and a liquid nitrogen cooled mercury-cadmium-telluride detector. A custom-built diffuse reflectance system with an IR-accessible gas dosing cell was used for all measurements. Sample temperature was controlled by an Oxford Instruments OptistatDry TLEX cryostat, and sample atmosphere was controlled by a Micromeritics ASAP 2020Plus gas sorption analyzer. In a typical experiment, a sample of the desolvated framework material was dispersed in dry KBr (10 wt. %) by gently mixing the two powders in an argon-filled glovebox and was subsequently evacuated at room temperature overnight. Spectra were collected in situ under UHP-grade 16 O 2 and 18 O 2 (99 atom % 18 O, Sigma-Aldrich) at 4 cm −1 resolution until equilibrium was observed in both pressure output and spectra. Peak fitting was performed in Origin using 2–4 Lorentzian peaks with the Levenberg-Marquardt algorithm. Spectra representative of various coverages with different superoxo species are shown (Supplementary Figs. 58 – 62 ). Hill equation analysis The occupancy values of the superoxo species, as determined by powder X-ray diffraction analysis, were fit to the Hill equation (Eq. 5 ), in which θ is the occupancy (between 0 and 1), [ L ] is the pressure of O 2 in bar, K d is the apparent dissociation constant, and n is the Hill coefficient, which can be approximately related to the number of binding sites [49] . It should be noted that we were unable to determine experimentally a physically-meaningful value for K d , so the parameter was allowed to freely refine in the process of all fits. θ = [L]^n/K_d + [L]^n
 (5) Additionally, in order to determine whether the adsorption of O 2 on the cobalt centers could be modeled to the Hill equation, the occupancies determined by X-ray powder diffraction were compared to the gas adsorption data. Stoichiometry, as well as X-ray powder diffraction analysis (detailed above) of the occupancy of reduced oxygen species within the pores of Co 2 (OH) 2 (bbta), reveal that the gas adsorption data encompasses both adsorption at coordinatively-unsaturated cobalt centers as well as physisorption. Low pressure adsorption data up to an unspecified regime should correspond to adsorption on isolated cobalt centers, whereas the occupancies determined from X-ray powder diffraction data could provide information about adsorption on the metal centers at high pressures, otherwise obscured by the large amount of physisorption in the gas adsorption data. In the X-ray powder diffraction data, in both the 7 mbar O 2 -dosed and 50 mbar O 2 -dosed Rietveld refinements, there is little evidence for occupancy of the physisorption site. These results indicate that the gas adsorption data up to at least 50 mbar is largely representative of metal-site adsorption. As a result of this assessment, the adsorption isotherm for O 2 in Co 2 (OH) 2 (bbta) at 195 K was fit between 0 bar and 0.05 bar with the Hill equation. It should be noted that the projected capacity values from the occupancies are slightly higher than the experimental gas adsorption capacities at low pressures, which may be due to defects (e.g. surface sites) that are not reflected in the occupancies. The fitting of the gas adsorption data for Co 2 Cl 2 (bbta) was also performed. In this instance, all values were unconstrained. We note, however, that when we constrain q sat to be the value expected for one O 2 per Co (5.77 mmol g −1 ), n and K d refine to be 1.30 and 0.85 respectively. These values result in greater deviations from the experimental points than the unconstrained values, and were ultimately disregarded, particularly as we could not justify a reason why n should be greater than 1. Rather, the saturation capacity of 16.9 mmol g −1 suggests that the unconstrained fitting might be reflective of pore-filling of the framework with O 2 , with 16.9 mmol g −1 being closer to the adsorption values that would be expected with an O 2 surface area at 90 K, rather than an interaction with the open metal site. This result is consistent with the X-ray powder diffraction and gas adsorption data that indicate a very weak interaction with O 2 . The residual sum of squares (“RSS”) and the average relative error (“ARE”) are reported with each associated fit. Measurements of d.c. magnetic susceptibility Samples were prepared by adding crystalline powder to a 5-mm i.d. 7-mm o.d. quartz tube containing a raised quartz platform. These samples include desolvated Co 2 Cl 2 (bbta) (9.8 mg), desolvated Co 2 (OH) 2 (bbta) (17.2 mg), methanol-solvated Co 2 (OH) 2 (bbta) (12.8 mg), Co 2 (OH) 2 (bbta) dosed with 0.5 equivalents of O 2 per cobalt (15.4 mg), and Co 2 (OH) 2 (bbta) dosed with 1 equivalent of O 2 per cobalt (11.4 mg). Sample powders were restrained with a plug of compacted glass wool that prevented crystallite torqueing, but enabled gas-dosing with O 2 . The methanol-solvated sample was filtered on a polypropylene membrane filter (0.45 μm) and dried briefly at room temperature under vacuum, before being loaded into the quartz tube. Air-free elemental analysis of the sample was measured on the same day of sample preparation in order to accurately quantify the amount of solvent adsorbed in the pores of the material. The O 2 -loaded samples were prepared by attaching the quartz tubes containing activated Co 2 (OH) 2 (bbta) to a Micromeritics ASAP 2020 gas adsorption analyzer. One equivalent of O 2 and 0.5 equivalents of O 2 for every Co atom within the structure was calculated and then exposed to the samples. All quartz tubes containing samples, including those loaded with O 2 gas, were flame-sealed while the sample was cooled with liquid nitrogen. Magnetic susceptibility measurements were performed using a Quantum Design MPMS2 SQUID magnetometer. Measurements of d.c. magnetic susceptibility were collected in the temperature range 2–300 K under applied magnetic fields of 1 T. Diamagnetic corrections were applied to the data using Pascal’s constants to give χ D = −0.00014552 emu mol −1 for desolvated Co 2 Cl 2 (bbta), χ D = −0.00011752 emu mol −1 for desolvated Co 2 (OH) 2 (bbta), χ D = −0.00019341 emu mol −1 for methanol-solvated Co 2 (OH) 2 (bbta), χ D = −0.00012672 emu mol −1 for Co 2 (OH) 2 (bbta) dosed with 0.5 equivalents of O 2 per cobalt, and χ D = −0.00013592 emu mol −1 for Co 2 (OH) 2 (bbta) dosed with 1 equivalent of O 2 per cobalt. The collected data is shown in Supplementary Figs. 63 – 65 . Theoretical calculations Periodic models for the desolvated and O 2 -loaded Co 2 Cl 2 (bbta) and Co 2 (OH) 2 (bbta) were optimized using the PBE-D3 functional [56] , [57] , as implemented in the VASP 5.4.4 program [58] . Dioxygen adsorption energies were obtained by single point calculations using the PBE0-D3 functional [59] with the PBE-D3 optimized structures. The vibrational properties were modeled using tetracobalt clusters, excised from the PBE-D3 optimized structures along a single helical chain. Constrained geometry optimizations were performed using the M06 [60] functional, where the dioxygen molecules, cobalt atoms, and the first coordination sphere of the two central cobalt atoms were allowed to relax. The electronic structure of the frameworks was evaluated using complete active space self-consistent field (CASSCF) single point calculations followed by second-order perturbation theory (CASPT2) using the MOLCAS 8.2 program [61] . An additional set of tetracobalt cluster models was employed, obtained from the experimental crystal structures of desolvated Co 2 Cl 2 (bbta) and Co 2 (OH) 2 (bbta). Dicobalt cluster models were obtained by replacing the external cobalt atoms by magnesium ions. Partial geometry optimizations were performed using the M06 functional by relaxing only C and H atoms. The computational details are further provided in the Supplementary Information. Markov chain simulations of negative cooperativity The framework metal sites were simulated, in a simplified fashion, as a chain of twelve Co atoms whose occupancies (bound or unbound to oxygen) at a given time were modeled as a Markov chain. At each time step, a random Co atom was chosen. If bound, the states of the Co atoms remained unchanged, reflecting the negligible probability of a bound Co atom becoming unbound in the timescales observed. If unbound, the chosen Co atom was changed to a bound state with a probability that decreased with the number of bound neighboring Co atoms, reflecting negative cooperativity. Periodic boundary conditions, simulating the repetition of such short chains in the material, were used to determine the neighbors of the first and last Co atoms. The Markov chain was run to T = 200 timesteps; the probability of an unbound Co atom becoming bound at any timestep given zero, one, and two bound neighbors was 0.5, 0.0005, and 0.0001, respectively. This data is shown in Supplementary Fig. 68 .